Low-energy electrodynamics of novel spin excitations in the quantum spin ice Yb2Ti2O7 In condensed matter systems, formation of long-range order (LRO) is often accompanied by new excitations. However, in many geometrically frustrated magnetic systems, conventional LRO is suppressed, while non-trivial spin correlations are still observed. A natural question to ask is then what is the nature of the excitations in this highly correlated state without broken symmetry? Frequently, applying a symmetry breaking field stabilizes excitations whose properties reflect certain aspects of the anomalous state without LRO. Here we report a THz spectroscopy study of novel excitations in quantum spin ice Yb 2 Ti 2 O 7 under a <001> directed magnetic field. At large positive fields, both right- and left-handed magnon and two-magnon-like excitations are observed. The g-factors of these excitations are dramatically enhanced in the low-field limit, showing a crossover of these states into features consistent with the quantum string-like excitations proposed to exist in quantum spin ice in small <001> fields. Geometrical frustration suppresses the formation of conventional long-range order (LRO) in magnetic materials to a temperature ( T C ) much lower than the Curie–Weiss temperature Θ CW (ref. 1 ). This provides the possibility of realizing novel states and excitations, as non-trivial spin correlations are often observed in these materials in the range T ≪ Θ CW even in the absence of LRO [2] . Magnetic pyrochlore oxides, in which magnetic rare earth ions sit at the vertices of corner-sharing tetrahedra, provide a fascinating material system in the search of such novel quantum ground states and excitations [3] . In spin ice materials such as Dy 2 Ti 2 O 7 and Ho 2 Ti 2 O 7 , strong crystal field anisotropy forces the spins to point along the local <111> direction, whereas long-range dipolar interaction between the spins provides an effective ferromagnetic interaction, giving a situation much resembling proton disorder in common water ice. Enforcing the ice rules in spin ice results in a ground state with each tetrahedron having the so-called ‘two-in, two-out’ configuration [4] , [5] . Flipping a single spin creates a pair of magnetic monopoles out of the ground-state vacuum in neighbouring tetrahedra, which can subsequently move away from each other through the network [6] , [7] . In applied field, a pair of magnetic monopoles with opposite magnetic charges are connected by a string of spins aligned against the field ( Fig. 1a ). Recent neutron scattering experiments have shown evidence for the existence of thermally activated Dirac strings and magnetic monopoles in classical spin ice materials [8] , [9] . 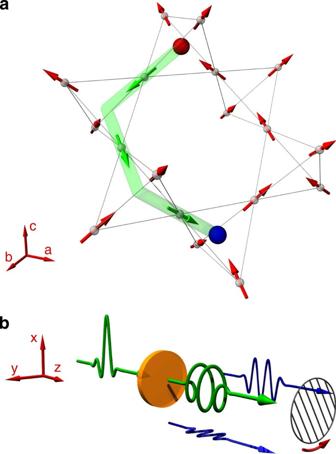Figure 1: Schematic of spin-ice and experimental setup. (a) Schematic illustration of a quantum string in <001> field in a pyrochlore spin ice. Monopole–antimonopole pairs are shown as red-blue spheres, spins with a negativezcomponent are shown as green arrows. Magnetic field is applied along thecdirection. (b) Schematic illustration of the experimental geometry. After a linearly polarized incident pulse passes through the sample, the two orthogonal components (ExandEy, shown as blue pulses) of the elliptically polarized transmitted pulse are measured with the polarimeter. The rotating wire grid polarizer shown in the figure is a key component of the polarimeter. Figure 1: Schematic of spin-ice and experimental setup. ( a ) Schematic illustration of a quantum string in <001> field in a pyrochlore spin ice. Monopole–antimonopole pairs are shown as red-blue spheres, spins with a negative z component are shown as green arrows. Magnetic field is applied along the c direction. ( b ) Schematic illustration of the experimental geometry. After a linearly polarized incident pulse passes through the sample, the two orthogonal components ( E x and E y , shown as blue pulses) of the elliptically polarized transmitted pulse are measured with the polarimeter. The rotating wire grid polarizer shown in the figure is a key component of the polarimeter. Full size image Recently, the material Yb 2 Ti 2 O 7 has attracted considerable attention [10] , [11] , [12] , [13] , [14] , [15] , [16] , [17] , [18] , [19] , [20] , [21] . Although the exact form of the low-temperature ground state is still under debate, the nature of the magnetic interactions place Yb 2 Ti 2 O 7 in the quantum spin ice regime. High-field inelastic neutron scattering (INS) experiments have obtained the exchange interaction parameters at low temperature, which demonstrates that in this material the ferromagnetic Ising-type exchange interaction is larger than the other terms in the Hamiltonian that lead to considerable quantum fluctuations and dynamics [14] . From considerations of crystal-field levels, its low-energy spin sector may be reduced to that of an effective spin-1/2 moment. A number of interesting effects have been proposed for this material, including it being a quantum spin liquid, whose elementary excitations carry fractional quantum numbers. Such a state supports an emergent quantum electrodynamics with a photon mode at low energy [22] , [23] , [24] . It was proposed recently that under weak applied <001> magnetic field (or in the presence of spontaneous magnetization), the elementary excitations of materials like Yb 2 Ti 2 O 7 take the form of extended ‘quantum strings’ consisting of fluctuating multiple flipped spins connecting monopole pairs [25] . With inherent quantum dynamics, these novel excitations are extended objects rather than point particles, an interesting feature of quantum spin ice. To explore the nature of the excitations in quantum spin ice, we performed time-domain terahertz spectroscopy (TDTS) measurements of Yb 2 Ti 2 O 7 single crystals under magnetic field applied along the <001> direction. Spectroscopic features consistent with the picture of quantum strings are observed in the low-field regime. When the field strength increases, a crossover towards field-induced order is observed where the excitations take the form of magnons and two-magnon excitations. Magneto-optical measurement Magneto-optical measurements are performed in a custom built time domain terahertz (THz) spectrometer. Two single crystals from the same travelling solvent floating zone boule are used in the measurement; they will be referred to as sample A and B throughout the text. The single-crystal Yb 2 Ti 2 O 7 samples are cut and polished with their surfaces oriented along the <001> plane. The sample is hosted in a 7-T superconducting magnet. Experiments are performed in transmission geometry as illustrated in Fig. 1b , with temperatures of the samples below the scale of the exchange interaction of Yb 2 Ti 2 O 7 . These temperatures are about one order of magnitude higher than the value of the debated ordering temperature T C , while at the same time low enough that spin correlations are well developed to allow the study of quantum spin ice physics. The incident THz pulse is linearly polarized, with the wavevector k of the pulse defining the z direction. Measurements are performed in both the Faraday geometry (applied magnetic field in the z direction) as well as the Voigt geometry (field in the y direction). In magnetic insulators, the complex transmission function we obtain is related to the complex frequency-dependent susceptibility χ( q =0) as −ln t ( ω ) ∝ ωχ( q =0, ω ) [26] . TDTS measures the q →0 response and as such is very useful for materials with interesting q =0 correlations [27] . The technique operates at a frequency range most relevant to the physics of quantum spin ice materials (0.4–10 meV); it has the strength of a high signal to noise ratio, excellent energy resolution and short acquisition times. Further details can be found in the Methods section. Magnetic excitations in Faraday geometry In the Faraday geometry, the applied static magnetic field is oriented along the THz pulse propagation direction, and the incident THz pulse is linearly polarized along the x axis of the laboratory frame. With the spins aligned and precessing around the applied field direction, one naturally expects magnetic absorption to be observed in the right circularly polarized (RCP) channel, which is a direct consequence of the fundamental coupling between magnetic field and spin precession. As a result, the magnetic excitations in this geometry would best be studied in the circular polarization frame, which can be measured with a phase-sensitive spectroscopic tool such as TDTS [28] , [29] , [30] , [31] (details can be found in the Methods section and Supplementary Notes 1 and 2 , as well as in the Supplementary Fig. 1 ). In Fig. 2a,b we show the transmission magnitude for the RCP and left circularly polarized (LCP) light as a function of frequency and field measured at 4.3 K from sample B in the Faraday geometry (see Methods for transformation to circular base). The measurements were taken every 0.5 T from 0 to 7 T. Clear dark lines diagonally across the figures immediately show the position of the absorptions in the spectra, revealing the existence of several branches of magnetic excitations. As we show in Supplementary Figs 2 and 3 , in this field range spectra taken at 1.65 and 4.3 K are almost identical, except that the absorptions are slightly sharper and stronger at 1.65 K. This demonstrates that we are in the low-temperature regime. Recalling that the quantity we explicitly measure (and are plotting) is proportional to ωχ ( q =0, ω ), we observe that these excitations are generally losing spectral weight in χ as the field increases and they move to higher ω . For the RCP channel, careful examination of the data reveals a total of five branches for fields higher than 3 T. They are labelled as b1, b2, b3, b5 , and b6 from low to high frequency. There is a single LCP branch, b4 , observed for fields higher than 4 T. This absorption in a +z magnetic field is anomalous and will be discussed in more detail below. Although branches b1 to b4 have similar slope in the frequency-field plot, suggesting similar effective g-factors, branches b5 and b6 clearly have higher g-factors. 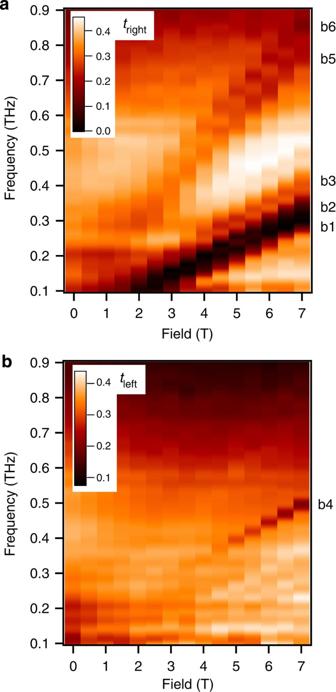Figure 2: Transmission measured in the Faraday geometry. (a,b) The intensity plot of the transmission of the (a) right circularly polarized light and (b) left circularly polarized light. Data presented here are measured from sample B at 4.3 K. Magnetic excitations are markedb1tob6from low to high frequency. Figure 2: Transmission measured in the Faraday geometry. ( a , b ) The intensity plot of the transmission of the ( a ) right circularly polarized light and ( b ) left circularly polarized light. Data presented here are measured from sample B at 4.3 K. Magnetic excitations are marked b1 to b6 from low to high frequency. Full size image In Yb 2 Ti 2 O 7 , there are four magnetic ions in each primitive unit cell; naively one would expect at most four spin waves modes, as has been observed in INS experiments recently [14] . The fact that six different branches of magnetic excitations are observed reveals the unconventional nature of some of these excitations. Another interesting feature is that as the observed excitations move to low frequencies at low field, they become less well defined and eventually turn into a broad magnetic absorption. Similar features are also obtained with sample A, from temperatures 1.65 K upward. All the features other than b1 and b2 fade away as temperature increases above 12 K. Details of the temperature dependence as well as additional data can be found in Supplementary Figs 2–6 , and relevant discussion in Supplementary Notes 3 and 4 . Magnetic excitations in Voigt geometry In the Voigt geometry, the magnetic field is oriented along the y direction. As a result, the circular frame is no longer an appropriate base for the study. Symmetry considerations dictate the absence of circular effects in this geometry [31] . Shown in Fig. 3a,b are the transmission magnitudes with electric polarization along the x direction, t xx , measured in sample A at 1.65 K, with Fig. 3b showing a more detailed measurement below 1 T, whereas results for t yy are shown in Fig. 3c . A total of four branches of magnetic excitations are observed, and labelled c1 to c4 from low to high frequency. Although c1 to c3 show similar g-factors, c4 shows a higher value. Excitations c2 and c4 show a notable downward concavity at low-magnetic fields. As will be discussed in detail below, we believe that these features are consistent with a picture of quantum spin ice where high-field one- and two-magnon states continuously evolve into string excitations at low field. 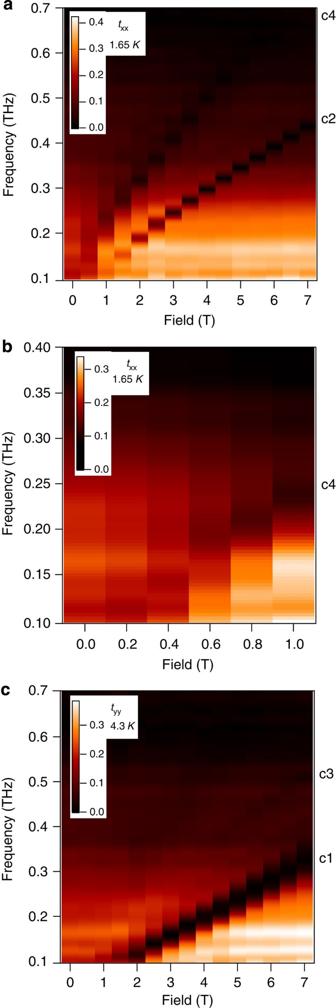Figure 3: Transmission as a function of field and frequency in Voigt geometry. Transmission magnitude as a function of frequency and field measured from sample A at 1.65 K with the electric polarization of the THz pulse in thexdirection (a,b), andydirection measured at 4.3 K (c). Foraandc, data were taken from 0 to 7 T with 0.5 T steps, andbshows the data below 1 T with 0.2 T steps. Magnetic excitations are labelledc1toc4from low to high frequency. Figure 3: Transmission as a function of field and frequency in Voigt geometry. Transmission magnitude as a function of frequency and field measured from sample A at 1.65 K with the electric polarization of the THz pulse in the x direction ( a , b ), and y direction measured at 4.3 K ( c ). For a and c , data were taken from 0 to 7 T with 0.5 T steps, and b shows the data below 1 T with 0.2 T steps. Magnetic excitations are labelled c1 to c4 from low to high frequency. Full size image As shown in Figs 2 and 3 , the magnetic excitations we observe at fields greater than 3 T in both the Faraday and Voigt geometries can be categorized into two groups: b1 to b4 and c1 to c3 having a similar, lower value of the g-factor (2.96–3.86, values listed in Fig. 4 caption), whereas b5 , b6 and c4 have larger g-factors (6.30–6.74). The frequencies of the observed magnetic excitations (with demagnetization correction applied) are summarized in Fig. 4a . 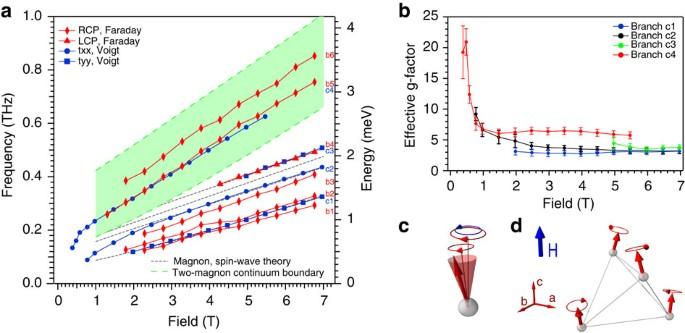Figure 4: Summary of the experimental and theoretical results. (a) Summary of the magnetic excitation frequencies as a function of field from both Faraday and Voigt geometries. Demagnetization correction has been applied to all the data shown in the figure. Experimental data are shown as solid symbols connected with lines, whereas dashed lines present results from theoretical calculations. All the data shown in the figure are measured at 1.65 K, except for thetyypolarization, which is taken at 4.3 K. Linear fits to data above 3 T yield the effective g-factors of the excitations to be:b1, b2andc1: 2.96;b3: 3.51;c2: 3.86;c3andb4: 3.72;c4: 6.30;b5: 6.56;b6, 6.74. (b) Effective g-factors taken from the slopes of branchesc1toc4measured from sample A at 1.65 K as a function of applied magnetic field. (c) Schematic illustration of the spin precession motion with a <001> applied field. For a single spin, the equilibrium direction will be slightly tilted away from the field direction. As a result, the precess motion has both a large clockwise component (red arrow) and a small counter-clockwise component (blue arrow) when viewed along the field direction. (d) When the four spins in a single tetrahedron all precess in phase, the resulting magnetic excitation is the observed magnon with the lowest energy with right circular polarization (b1, b2, c1). Figure 4: Summary of the experimental and theoretical results. ( a ) Summary of the magnetic excitation frequencies as a function of field from both Faraday and Voigt geometries. Demagnetization correction has been applied to all the data shown in the figure. Experimental data are shown as solid symbols connected with lines, whereas dashed lines present results from theoretical calculations. All the data shown in the figure are measured at 1.65 K, except for the t yy polarization, which is taken at 4.3 K. Linear fits to data above 3 T yield the effective g-factors of the excitations to be: b1, b2 and c1 : 2.96; b3 : 3.51; c2 : 3.86; c3 and b4 : 3.72; c4 : 6.30; b5 : 6.56; b6 , 6.74. ( b ) Effective g-factors taken from the slopes of branches c1 to c4 measured from sample A at 1.65 K as a function of applied magnetic field. ( c ) Schematic illustration of the spin precession motion with a <001> applied field. For a single spin, the equilibrium direction will be slightly tilted away from the field direction. As a result, the precess motion has both a large clockwise component (red arrow) and a small counter-clockwise component (blue arrow) when viewed along the field direction. ( d ) When the four spins in a single tetrahedron all precess in phase, the resulting magnetic excitation is the observed magnon with the lowest energy with right circular polarization ( b1, b2, c1 ). Full size image Upon examination of the complete data set, one notices that the energies of the magnetic excitations with lower g-factors are in the same range as the magnons observed by INS in the field-induced ordered state of Yb 2 Ti 2 O 7 (ref. 14 ). Although the direction of the applied magnetic field in the INS experiment is different from the present study, this provides a useful hint in establishing the nature of those branches of excitations observed in our TDTS as magnons. To form a better understanding of the observed magnetic excitations, we performed a spin-wave analysis with the interaction parameters obtained in ref. 14 as the starting point. Linear spin-wave theory predicts a total of four magnon modes, given the four unique spins in the unit cell of Yb 2 Ti 2 O 7 . Only two of the magnon modes are predicted to be visible as q →0 in the Faraday geometry, whereas in the Voigt geometry three modes are predicted to be visible. As shown in Fig. 4 , both the energy and the polarization state of the excitations observed in the LCP in the Faraday geometry as well as the ones in the Voigt geometry match the spin-wave theory prediction very well at high fields, where the field-induced LRO supports the existence of well-defined magnon modes. With the high signal-to-noise ratio of the TDTS, the data above 3 T from these three branches allowed a further refinement of the exchange parameters in a least squares fitting procedure (see Supplementary Note 5 for further details). One surprising aspect of the data was the clear observation of a LCP branch b4 when the magnetic field was applied in the +z direction ( Fig. 2b ). As mentioned above, at first sight this seems to be in contradiction to the natural coupling between magnetic field and spin moments. Previously such LCP spin precession has only been proposed for metallic ferromagnets with strong spin-orbit interaction [32] . This interesting observation finds a natural explanation in the context of the spin-wave theory. With the easy plane anisotropy of the Yb 3+ ion, the equilibrium direction of the spin is tilted away from the <001> axis, moreover, the spin precession is slightly elliptical around the applied field in the <001> direction. Thus, the precession motion has both LCP and RCP components when viewed along the field direction. This is schematically illustrated in Fig. 4c,d . For the highest-energy magnon mode, which corresponds to the b4 / c3 branches, the phase relationship between the spins in the unit cell is such that the RCP components cancel exactly, leaving only the LCP component in the Faraday geometry. Another interesting feature of the data is the observation of excitations with clearly higher g-factors than the magnons. A closer examination of the data reveals that excitations b5 , b6 and c4 have a g-factor about twice the value of the magnon branches. Interestingly, they also appear in the middle of the two-magnon continuum band obtained from the spin-wave calculation, as shown in Fig. 4a . These suggest that although the branches b1 to b4 and c1 to c3 can be understood as magnons, b5 , b6 and c4 are two-magnon excitations. The fact that they appear in the middle of the calculated two-magnon continuum, suggests they are unlikely to be simple two-magnon bound states. Thus, it remains to be understood how these excitations can be stable and have well-defined energies. Moreover, our spin-wave calculations show that these excitations do not match any peaks in the joint two-magnon density of states (details of the calculation are provided in Supplementary Notes 5 and 6 , a comparison of calculation and experimental data can be found in Supplementary Fig. 7 ). Note that the two-magnon continuum band intersects with the single-magnon modes at low fields. This gives the possibility of decay for the higher energy single magnons at low fields. Also at odds with the spin-wave calculation is the observation of four single magnon-like branches in the Faraday geometry, as only the highest and the lowest modes are expected to be visible. In comparing the geometries, b1 , b2 , and c1 all appear in the energy range of the calculated lowest magnon mode. Our data suggest that b1 and b2 are distinct features (more clearly shown in Supplementary Figs 1 and 5 ), although they are difficult to distinguish because of the strong absorption in this frequency range. They may derive from the same lowest-energy magnon state, but with some unexplained splitting. Moreover, it is difficult to understand b3 as the second or third highest magnons that have picked up a finite intensity by some means (from misalignment of the applied field for instance). Its energy is below the c2 excitation in the Voigt geometry, which is straightforwardly assigned to the second highest magnon mode. These discrepancies that appear only in the Faraday geometry are as of yet unexplained. Further details of the spin-wave analysis of the four magnon modes are given in Supplementary Notes 5 and 6 . As field decreases, the match between the spin-wave calculation and the experiments becomes progressively worse ( Fig. 4a ). At the temperature range of the study, spin correlations are well developed and at low fields the material approaches the nominal quantum spin ice regime [12] , [33] . Thus, it is not surprising to see the spin-wave theory fails at low fields. The spectroscopic features in this region reveal the nature of the excitations unique to the quantum spin ice state. Among those features, the most prominent one is the change of slope of the magnetic excitations at low fields. We believe this large concave downward non-linearity is a general signature of quantum mixing of states with different numbers of spin flips. When the field is lowered from the high-field regime (where the excitations should be understood as spin flips of a quantized number, for example, magnons), the excitations of the system are now expected to be admixtures of chains of flipped spins with different lengths, as proposed in the quantum string picture and also observed in spin chains [34] . In this scenario, one expects that as the field diminishes, strings get longer. As a result, their g-factor increases and the slope of the curve goes up. The strong enhancement of these g-factors below 2 T clearly observed for branches c2 and c4 as field decreases provides strong support for this picture, as shown in Fig. 4b . This strong increase of g-factors is evidence of significant admixing of states of many flipped spins in this part of the phase diagram. We should point out that although ferromagnetic resonance can give qualitatively similar field dependences, such a scenario requires ferromagnetic order, which is obviously not present here. The quantum string picture was derived with the assumption that both the transverse exchange and magnetic field B are small compared with the diagonal Ising exchange [25] . It requires the breaking of time-reversal symmetry either by a <001> directed field or by a spontaneous magnetization in this direction. As shown here and elsewhere [14] , transverse exchange terms are not small in the material Yb 2 Ti 2 O 7 , but it was argued in ref. 25 that as long as the regime of interest was adiabatically connected to the perturbative regime, the qualitative string picture should be robust. It was proposed that a hierarchy of states would be observed corresponding to strings of different lengths. However, in real materials with multiple spins in the unit cell and finite non-Ising transverse exchange terms, a hierarchy of states might be difficult to realize explicitly because of the decay channels opening up with overlapping bands of multi-string and multi-magnon continuums (as implied in Fig. 4a ). In the present study, high-field two-magnon excitations are observed to evolve continuously into string states at low fields, although their stability remains to be understood. In any case, one may still expect that the lowest magnon features observed at high fields evolve into string-like states at low fields. Our observations are consistent with such a picture that the lowest elementary excitations of a quantum spin ice in small magnetic fields are quantum strings connecting weakly bound monopoles. As discussed above, the application of a symmetry breaking field can stabilize excitations whose properties reflect certain aspects of an anomalous state without LRO. In the present case, the observation of a crossover from magnons to strings as the field is decreased reflects the presence of deconfined monopoles in the zero-field quantum spin ice state. Sample fabrication and characterization Single-crystal samples of Yb 2 Ti 2 O 7 were grown at McMaster University with the optical floating zone technique. Details of the sample growth are discussed elsewhere [17] . Samples A and B used for the THz measurements are two single crystals with their largest surface oriented parallel to the <001> plane. Sample A has a circular cross-section with a diameter of 4.2 mm, with thickness of 0.725 mm, whereas sample B has a rectangular cross-section that measures 5.46 by 2.37 mm, with a thickness of 0.648 mm. Both samples are transparent. Laue X-ray diffraction was performed to assure the samples used do not contain domains of misaligned microstructure or crystallites. The low-temperature heat capacity of sample B has been measured from 150 to 800 mK, and shows the same behaviour as the non-annealed crystal reported in ref. 17 . As shown in refs 33 and 35 , at temperatures of our current study, the exact nature of the low-temperature ground state is not relevant, as the entire phase diagram is predicted to be in the thermal spin liquid state at temperatures just below the scale of J zz . Also, as reported in refs 17 , 20 and 21 , sample variations are minimal for temperatures above 1 K, thus the possible sample variation does not affect our conclusion in this paper. Time domain terahertz spectrometer setup A home-built TDTS was set up at Johns Hopkins University with two dipole switches as THz emitter and receiver. The sample was hosted in a cryogen-free split coil superconducting magnet. The magnet provides magnetic fields up to 7 T, and a base temperature down to 1.6 K for the measurements. The magnet has four windows allowing for optical access, and can be switched between Faraday and Voigt geometries. The single-crystal samples were mounted on a metal aperture. The electric field profiles of the terahertz pulses transmitted through the sample and an identical bare aperture were recorded as a function of delay stage position, and then converted to time traces. Fast Fourier Transforms (FFTs) of the sample and aperture scans gave the complex transmitted and incident pulse spectra, from which the complex transmission coefficients were obtained. Polarization modulation technique in terahertz polarimeter As shown in the previous sections, the simultaneous measurement of two orthogonal components of the transmitted THz pulse is critical for this experiment. This is realized by a terahertz polarimeter with polarization modulation technique based on a rotating polarizer developed recently [28] . The main setup contains three polarizers, one rotates at angular velocity Ω that modulates the polarization state of the THz pulse to be measured (shown in Fig. 1b ); a second one downstream oriented with the transmission axis parallel to the x axis. Another polarizer upstream creates a linearly polarized incident pulse before the sample. The effect of the two polarizers in the polarimeter on an arbitrary electric field vector can be expressed as a product of two matrices: where: straightforward algebra gives: Here Θ=Ωt+ Φ is the angle of the rotating polarizer with respect to the x axis, Φ 0 is the initial angle. The signal detected after the polarimeter is then fed into a lock-in amplifier with a reference signal of frequency 2Ω. In this way, the in-phase and out-of-phase readings of the lock-in amplifier measure and simultaneously, with an appropriate choice of Φ 0 . Note that it is important that the sense of rotation (direction of the angular velocity Ω) of the rotating polarizer be the same as the THz pulse propagation direction; otherwise instead of , will be measured, which would give a reversed definition of right/left circular polarization. See ref. 25 for further details on this technique. Transforming into circular base in the Faraday geometry Following the previous section, when and of the transmitted pulse are measured while retaining their phases, it is possible to transform the frame of reference into circular polarized frame, thus providing an opportunity to study the magnetic excitations in their natural circularly polarized basis in the Faraday geometry. With , standing for the electric field component in RCP and LCP channels, we have: More details of this transformation of bases can be found in Supplementary Notes 1 and 2 . How to cite this article: Pan, L. D. et al . Low-energy electrodynamics of novel spin excitations in the quantum spin ice Yb 2 Ti 2 O 7 . Nat. Commun. 5:4970 doi: 10.1038/ncomms5970 (2014).